Fudging the volcano-plot without dredging the data While the fudge factor was originally introduced as a small positive constant (denoted as \({s}_{0}\) ) to improve the independence of the test statistic variance and of the omic feature expression, its tuning to a larger value has been observed to yield a user-defined weighting of the significance and of the effect size. Concomitantly, the permutation-based procedure of SAM test has sometimes been replaced by classical p-value adjustment –as prescribed in the Benjamini-Hochberg (BH) procedure for FDR control [5] . Applying simultaneously these two tricks enhances volcano-plot interpretation: the biomarkers selected are located in the outer spray of the volcano-plot, with selection boundaries following hyperbolic contours (see Fig. 1 ). Unfortunately doing so jeopardizes the statistical guarantees: briefly, a too large \({s}_{0}\) value distorts the p-values as well as the subsequent adjusted p-values calculated in the BH procedure. To cope with this, it is either necessary to constrain the tuning of \({s}_{0}\) (at the cost of less flexible selection of the outer spray) or to replace BH procedure by another FDR control method that does not require any p-value adjustment. 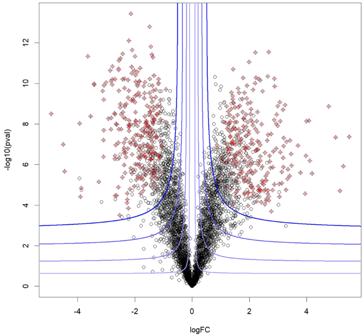Fig. 1: A typical volcano-plot. A significance measure is depicted on the Y-axis (here, -log10(p-value)) and an effect size is depicted on the X-axis (here, the logarithmized fold-change). The blue lines represent the contours of the relevance score and the points highlighted in red are those selected according to a knockoff procedure. Although the permutation-based procedure associated to SAM test is an option, it does not strictly controls for the FDR (see Table 1 ). Bayer et al. have thus explored another option inspired by TDC, which has emerged nearly twenty years ago in proteomics in absence of p-values to assess the significance of peptide identification. Fig. 1: A typical volcano-plot. A significance measure is depicted on the Y-axis (here, -log10(p-value)) and an effect size is depicted on the X-axis (here, the logarithmized fold-change). The blue lines represent the contours of the relevance score and the points highlighted in red are those selected according to a knockoff procedure. Full size image Table 1 Pros and cons of the various approach to FDR control with respect to selecting biomarkers on the outer spray of the volcano-plot Full size table Although published a decade later, the most convincing theoretical support of TDC to date has been knock-off filters (or KO) [6] , [7] . In spite of minor discrepancies with TDC [8] , KO mathematically justifies TDC general approach to FDR control, as well as its main computational steps. Notably, it demonstrates that FDR can be controlled on a biomarker selection task by thresholding a contrast of relevance scores, which results from a pairwise competition between the real putative biomarkers and other ones, fictionalized –respectively referred to as decoys and knock-offs in the proteomic and statistic parlances. Intuitively, the proportion of fictionalized features selected should be a decent proxy of the ratio of false discoveries [ Nota Bene : In KO theory, this proportion is corrected by adding 1 to the ratio numerator to cope for a bias issue. Although this bias is still investigated [9] , this suggests to correct for Eq. 16 in [1] by adding 1 to the numerator too. ], as long as the decision is made symmetrically ( i.e .﻿,﻿ their relevance score is attributed regardless of their real/fictional status). However, despite conceptual similarities, the problems solvable by TDC and KO differ: For the former, features are classically amino acid sequences; while for the latter, a quantitative dataset describing biomolecular expression levels in response to various experimental conditions is classically considered. In this context, the TDC extension proposed in CurveCurator to process quantitative dose-response curves constitutes a nice bridge between the TDC and KO kingdoms. With this in mind, the pragmatic fallouts of Bayer et al. become striking. Any data analyst wishing to select omic biomarkers with a relevance score picturing hyperbolic contours on a volcano plot (see Fig. 1 ) can easily adapt CurveCurator approach to their own case, by following the above procedure: (1) Perform statistical tests to obtain a p-value for each putative biomarker that assess the significance of its differential status, (2) Likewise, compute the biomarker fold-change, as a measure of the effect size, and construct the volcano-plot, (3) Tune \({s}_{0}\) to blend the significance of the differential status and the effect size into a single relevance score, (4) Acknowledge the relevance score looks like a p-value even though it may not be valid to use it as such, depending on the \({s}_{0}\) chosen, (5) Rely on the KO framework ( e.g ., using the “knockoff” R package ( https://cran.r-project.org/web/packages/knockoff/index.html ) as well as on the numerous tutorials available ( https://web.stanford.edu/group/candes/knockoffs/software/knockoffs/ ) to control for the FDR on the biomarker selected according to the relevance score, in a way similar to that of CurveCurator. An important and possibly troublesome feature of Fig. 1 is that some “unselected” black points are surrounded by “selected” red ones. In other words, some putative biomarkers may not be retained while other ones with smaller effect size and larger raw p-value are. This is a classical drawback of competition-based FDR control methods: each putative biomarker being retained or not does not only depend on its features, but also on those of its fictionalized counterpart, which generation is subject to randomness. Although this weakness can be addressed too, it requires less straightforward tools [10] . Another still open problem in KO theory lies in the KO/decoy generation, which can be difficult depending on the dataset. With this respect, the approach of CurveCurator is worthwhile. More generally, no method is perfect: KO filters, like p-value adjustment or permutation-based control have pros and cons (see Table 1 ). Therefore, depending on the data analyst ‘need, the preferred method should change. Considering this need for multiple off-the-shelf tools, it is important to notice that KO filters have hardly spread beyond the theoretical community so far, and that their applications to enhance data analysis in biology-centered investigations are still scarce, unfortunately. In this context, the seminal proposal of Bayer et al. can be expected to foster the translation of these fast-evolving theories into practical and efficient software with growing importance in biomarker discoveries, and they must be acknowledged for this.